Phosphatidylinositol(4,5)bisphosphate coordinates actin-mediated mobilization and translocation of secretory vesicles to the plasma membrane of chromaffin cells Neurosecretory vesicles undergo docking and priming before Ca 2+ -dependent fusion with the plasma membrane. Although de novo synthesis of phosphatidylinositol(4,5)bisphosphate (PtdIns(4,5) P 2 ) is required for exocytosis, its precise contribution is still unclear. Here we show that inhibition of the p110δ isoform of PI3-kinase by IC87114 promotes a transient increase in PtdIns(4,5) P 2 , leading to a potentiation of exocytosis in chromaffin cells. We then exploit this pathway to examine the effect of a transient PtdIns(4,5) P 2 increase on neurosecretory vesicles behaviour, outside the context of a secretagogue stimulation. Our results demonstrate that a rise in PtdIns(4,5) P 2 is sufficient to promote the mobilization and recruitment of secretory vesicles to the plasma membrane via Cdc42-mediated actin reorganization. PtdIns(4,5) P 2 , therefore, orchestrates the actin-based conveyance of secretory vesicles to the plasma membrane. Neuronal and hormonal communication relies on the regulated release of neurotransmitters stored in secretory vesicles through a process known as exocytosis. In chromaffin cells, most vesicles are separated from the plasma membrane by a dense cortical network of actin filaments. Following stimulation of exocytosis this restrictive barrier is disrupted, allowing vesicles to translocate to the plasma membrane and undergo fusion [1] . Such disruption is initiated by Ca 2+ and mediated by proteins such as scinderin [1] and MARCKS [2] . A more active role for actin during vesicle exocytosis has recently been suggested [3] . Phosphoinositides have a critical role in exocytosis [4] , [5] , [6] , [7] , [8] , [9] , [10] , [11] . First, manipulation of phospholipase C activity affects exocytosis [5] . Second, phosphatidylinositol transfer protein (PITPα) and phosphatidylinositol 4-phosphate 5-kinase (PI4P5K) are essential for ATP-dependent priming [6] . Third, PtdIns(4,5) P 2 sequestration by the Phospholipase C δ 1 Pleckstrin homology domain (PH-PLCδ 1 ) domain or redistribution of PtdIns(4,5) P 2 to endocytic organelles by expression of a constitutively active ARF6 mutant inhibits secretion [4] , [7] . Fourth, intracellular application of PtdIns(4,5) P 2 increases the size of the readily releasable pools in pancreatic β cells, and neutralization of a PtdIns(4,5) P 2 effector, Ca 2+ -dependent activator protein for secretion (CAPS), also abolishes secretion [12] . Finally, manipulation of PtdIns(4,5) P 2 levels using a pan-PI3-kinase (PI3K) inhibitor has revealed that PtdIns(4,5) P 2 controls the readily releasable pool of secretory vesicles [8] . These lines of evidence point to a role for PtdIns(4,5) P 2 in mediating ATP-dependent priming, which is known to be a relatively early event in exocytosis. Our current knowledge of PtdIns(4,5) P 2 effectors is mainly restricted to the latest steps of exocytosis [13] . However, a number of additional PtdIns(4,5) P 2 effectors, including CAPS [14] , are likely to act during the priming stage. De novo synthesis of PtdIns(4,5) P 2 is a critical step in the ATP-dependent priming that occurs following stimulation of exocytosis [6] . One of the key issues in understanding the role of PtdIns(4,5) P 2 in secretion is that it has not yet been possible to dissect its actual contribution in isolation from the context of secretagogue stimulation. Short-term application of the pan PI3-kinase inhibitor LY294002 has been shown to elicit a transient increase in PtdIns(4,5) P 2 that correlates with a potentiation of secretion [8] . Such PtdIns(4,5) P 2 was detected in isolated plasma membrane sheets from chromaffin cells in the absence of Ca 2+ and cytosol, suggesting that the machinery responsible for PtdIns(4,5) P 2 synthesis could be present on the plasma membrane. To investigate this contribution, we characterized the nature of this PI3K-sensitive and cytosol-independent pathway and then exploited it to investigate the role of PtdIns(4,5) P 2 in exocytosis. Our results reveal that the increase in PtdIns(4,5) P 2 elicited through pharmacological inhibition of class I PI3Kδ is sufficient to promote Cdc42-mediated actin reorganization that allows the translocation of secretory granules towards the plasma membrane. Inhibition of PI3Kδ by IC87114 potentiates exocytosis PtdIns(4,5) P 2 levels have been reported to transiently increase in response to treatment with LY294002, a broad-spectrum PI3K inhibitor [8] . Although this effect correlated with an increase in secretion, the actual contribution of PI3K remained unclear [15] 15. We hypothesize that LY294002 could promote a transient increase in PtdIns(4,5) P 2 levels via perturbation of the dynamic equilibrium between PtdIns(4,5) P 2 and PtdIns(3,4,5) P 3 controlled by a class I PI3K and the 3-phosphatase PTEN. The recent development of isoform-selective class I PI3K inhibitors allowed us to test the possible contribution of this class of enzymes to exocytosis, and their possible contribution to PtdIns(4,5) P 2 production. Cultured bovine chromaffin cells were incubated with increasing concentrations of isoform-specific inhibitors for PI3Kβ (TGX-221) [16] , PI3Kδ (IC87114) [17] or PI3Kγ (AS252424) [18] and briefly stimulated using barium chloride (Ba 2+ ) in the continuing presence of inhibitors ( Fig. 1a–c ). IC87114, a potent inhibitor of PI3Kδ, had a potentiating effect on Ba 2+ -stimulated catecholamine release from chromaffin cells ( Fig. 1b ). Interestingly, this was observed with as little as 1 min of IC87114 preincubation ( Fig. 1d ). In the absence of secretagogue, IC87114 had no effect on basal catecholamine release ( Fig. 1e ). We hypothesized that IC87114-mediated potentiation of exocytosis was promoted by a local increase in PtdIns(4,5) P 2 and should therefore be independent of the type of voltage-gated Ca 2+ channels activated by the secretagogue. To bypass Ca 2+ channels, digitonin-permeabilized chromaffin cells were incubated with increasing concentrations of IC87114 before stimulation with EGTA-buffered Ca 2+ . Under these conditions, IC87114-induced potentiation was still apparent ( Fig. 1f ). We also demonstrated that IC87114 did not affect activity-dependent Ca 2+ influx in chromaffin cells loaded with the Ca 2+ indicator Fluo4/AM ( Supplementary Fig. S1 ). 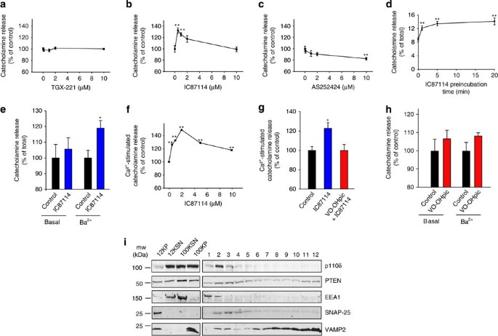Figure 1: Effect of isoform-selective PI3K inhibitors on catecholamine release from chromaffin cells. Cultured bovine chromaffin cells were briefly washed with buffer A and incubated with increasing concentrations of (a) TGX-221 (b) IC87114 or (c) AS252424 before being further stimulated using barium chloride (2 mM) for 2 min in the continuing presence of inhibitors. (d) Chromaffin cells were treated with IC87114 (1 μM) for the indicated time period before being stimulated using barium chloride (2 mM) for 2 min. (e) Chromaffin cells were incubated with or without IC87114 for 20 min before being stimulated using barium chloride (2 mM) for 2 min. (f) Chromaffin cells were treated with the indicated concentrations of IC87114 for 5 min before stimulation using digitonin (20 μM) permeabilization in the presence of 10 μM Ca2+and 2 mM MgATP in KGEP buffer. (g) Chromaffin cells were pre-incubated with or without VO-OHpic (100 nM) in buffer A before the addition of IC87114 (1 μM). Cells were then stimulated as described above. (h) Chromaffin cells were pre-treated with VO-OHpic (100 nM) before being stimulated using barium chloride (2 mM) for 2 min. Aliquots of the supernatant were removed and assayed fluorimetrically for catecholamine content. Data are expressed as mean±s.e.m.n=8, **Student'st-test,P<0.01, representative experiments carried out at least 4 times in octuplicate. (i) Subcellular fractions were prepared from bovine adrenal medulla (12KP and 12KSN=pellet and supernatant from 12,000gavspin; 100KP and 100KSN=pellet and supernatant from the 100,000gavspin). The chromaffin granule-containing 12KP fraction was loaded on a linear sucrose gradient (1M–2.2M) and fractions collected from the top (1–12). 50 μg protein from each fraction were separated and analysed by SDS–PAGE and western blotting using the indicated antibodies. The position of the early endosome, plasma membrane and secretory granules containing fractions was detected using anti-EEA1, anti-SNAP-25 and anti-VAMP2 antibodies, respectively. Figure 1: Effect of isoform-selective PI3K inhibitors on catecholamine release from chromaffin cells. Cultured bovine chromaffin cells were briefly washed with buffer A and incubated with increasing concentrations of ( a ) TGX-221 ( b ) IC87114 or ( c ) AS252424 before being further stimulated using barium chloride (2 mM) for 2 min in the continuing presence of inhibitors. ( d ) Chromaffin cells were treated with IC87114 (1 μM) for the indicated time period before being stimulated using barium chloride (2 mM) for 2 min. ( e ) Chromaffin cells were incubated with or without IC87114 for 20 min before being stimulated using barium chloride (2 mM) for 2 min. ( f ) Chromaffin cells were treated with the indicated concentrations of IC87114 for 5 min before stimulation using digitonin (20 μM) permeabilization in the presence of 10 μM Ca 2+ and 2 mM MgATP in KGEP buffer. ( g ) Chromaffin cells were pre-incubated with or without VO-OHpic (100 nM) in buffer A before the addition of IC87114 (1 μM). Cells were then stimulated as described above. ( h ) Chromaffin cells were pre-treated with VO-OHpic (100 nM) before being stimulated using barium chloride (2 mM) for 2 min. Aliquots of the supernatant were removed and assayed fluorimetrically for catecholamine content. Data are expressed as mean±s.e.m. n =8, **Student's t -test, P <0.01, representative experiments carried out at least 4 times in octuplicate. ( i ) Subcellular fractions were prepared from bovine adrenal medulla (12KP and 12KSN=pellet and supernatant from 12,000 g av spin; 100KP and 100KSN=pellet and supernatant from the 100,000 g av spin). The chromaffin granule-containing 12KP fraction was loaded on a linear sucrose gradient (1M–2.2M) and fractions collected from the top (1–12). 50 μg protein from each fraction were separated and analysed by SDS–PAGE and western blotting using the indicated antibodies. The position of the early endosome, plasma membrane and secretory granules containing fractions was detected using anti-EEA1, anti-SNAP-25 and anti-VAMP2 antibodies, respectively. Full size image PI3Kδ has recently been shown to negatively regulate the 3-phosphatase PTEN [19] . In response to IC87114, the dynamic equilibrium between PtdIns(4,5) P 2 and PtdIns(3,4,5) P 3 should therefore be shifted towards PtdIns(4,5) P 2 through the increased activity of PTEN leading to a transient rise in PtdIns(4,5) P 2 . We tested this hypothesis by preincubating chromaffin cells with VO-OHpic, a PTEN-specific inhibitor [20] . Whereas IC87114 promoted a significant potentiation of Ca 2+ -stimulated catecholamine release from digitonin-permeabilized chromaffin cells ( Fig. 1g ), preincubating cells with VO-OHpic abolished this effect ( Fig. 1e ). Importantly, VO-OHpic treatment alone had no effect on basal or Ba 2+ -stimulated release ( Fig. 1h ). These data suggest that PI3Kδ inhibition potentiates exocytosis by increasing PtdIns(4,5) P 2 levels not only by preventing production of PtdIns(3,4,5) P 3 by PI3Kδ, but also through the dephosphorylation of PtdIns(3,4,5) P 3 by the disinhibited PTEN. PI3Kδ and PTEN are expressed in chromaffin cells Recent evidence has shown that PI3Kδ is highly expressed in the central nervous system [21] . To determine whether PI3Kδ and PTEN are also expressed in chromaffin cells, we performed a subcellular fractionation and found that both proteins were present in both the cytosol and membrane fractions of these cells ( Fig. 1i ). p110δ, the catalytic subunit of PI3Kδ, was restricted to light membranes (100KP and fraction 2) whereas PTEN had a broader distribution, with a first peak similar to that of SNAP-25 (synaptosome-associated protein of 25,000 daltons), a plasma membrane marker, and a second peak corresponding to the heavy membrane-containing fractions 11 and 12 that are enriched for the secretory granule marker, vesicle-associated membrane protein (VAMP2) ( Fig. 1i ). This suggests that a pool of PI3Kδ and PTEN is present on the plasma membrane, as previously suggested [22] , and that an extra pool of PTEN may also be present on secretory vesicles. p110δ inhibition by IC87114 increases PtdIns(4,5) P 2 levels Our experiments pointed to a role for PI3Kδ in regulating PtdIns(4,5) P 2 synthesis and exocytosis. To further test this idea, we isolated chromaffin cells from wild-type and mutant knock-in–knockout mice in which both p110δ alleles have been replaced by a kinase-dead mutant p110 D910A/D910A [23] . Both wild-type and mutant cell types were treated with IC87114 and the level of PtdIns(4,5) P 2 analysed by thin layer chromatography (TLC) followed by an overlay assay using the PtdIns(4,5) P 2 -specific antibody 2C11 (ref. 24 ). IC87114 promoted a significant increase in PtdIns(4,5) P 2 in the wild-type cells ( Fig. 2a ), but not in the mutant cells ( Fig. 2b ). Chromaffin cells extracted from the mutant mice had slightly less PtdIns(4,5) P 2 , although this was not statistically significant ( Supplementary Fig. S2 ). 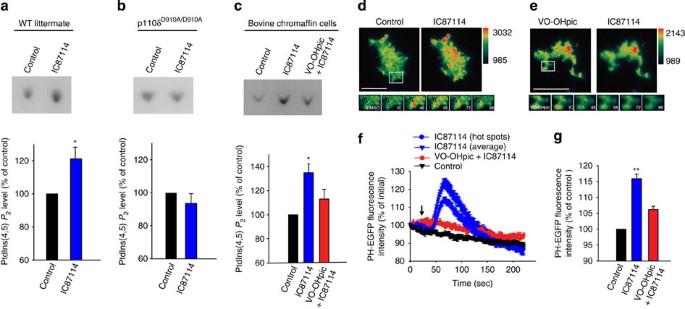Figure 2: IC87114-induced increase in PtdIns(4,5)P2levels is specific to PI3Kδ and dependent on PTEN activity. Mouse chromaffin cells were isolated from (a) wild-type (WT) littermate or (b) p110 δD910A/D910Amutant mice and treated with vehicle or IC87114 (1 μM) for 5 min before extracting phosphoinositides with acidified chloroform:methanol extraction and probing for PtdIns(4,5)P2using the anti-PtdIns(4,5)P2antibody, 2C11. Representative TLC blots from 4–6 independent experiments are shown. (c) Cultured bovine chromaffin cells were pre-incubated with or without VO-OHpic (100 nM) in buffer A for 20 min and subsequently treated for 5 min with vehicle alone or IC87114 (1 μM). Phosphoinositides were extracted as described above and PtdIns(4,5)P2levels detected using the 2C11 antibody. A representative example of a TLC blot from 3 independent experiments is shown. Quantification of the change in PtdIns(4,5)P2levels was achieved by densitometry analysis as described in the Methods section, and values are expressed as mean±s.e.m. (n=6 for WT,n=4 for p110 δD910A/D910A,n=3 for bovine chromaffin cells, Student'st-test, *P<0.05). (d,e) Chromaffin cells were transfected with PH-PLCδ1-EGFP, and plasma membrane patches were examined by TIRF microscopy at 1 frame per second. Images are displayed in pseudocolour to highlight the changes in fluorescence intensity in the indicated conditions. The images shown were taken from the beginning (left) and peak (right) of the IC87114-induced effect. The insets display the fluorescence intensity change from a selected region of interest on the plasma membrane patches taken at the indicated time points. (f) Time-course variation of PH-PLCδ1-EGFP fluorescence intensity on the (selected) plasma membrane patches in the indicated conditions. (g) Average peak fluorescence intensity change of PH-PLCδ1-EGFP in the respective conditions expressed as mean±s.e.m. (Student'st-test, **P<0.01). Scale bar, 10 μm. Figure 2: IC87114-induced increase in PtdIns(4,5)P 2 levels is specific to PI3Kδ and dependent on PTEN activity. Mouse chromaffin cells were isolated from ( a ) wild-type (WT) littermate or ( b ) p110 δ D910A/D910A mutant mice and treated with vehicle or IC87114 (1 μM) for 5 min before extracting phosphoinositides with acidified chloroform:methanol extraction and probing for PtdIns(4,5) P 2 using the anti-PtdIns(4,5) P 2 antibody, 2C11. Representative TLC blots from 4–6 independent experiments are shown. ( c ) Cultured bovine chromaffin cells were pre-incubated with or without VO-OHpic (100 nM) in buffer A for 20 min and subsequently treated for 5 min with vehicle alone or IC87114 (1 μM). Phosphoinositides were extracted as described above and PtdIns(4,5) P 2 levels detected using the 2C11 antibody. A representative example of a TLC blot from 3 independent experiments is shown. Quantification of the change in PtdIns(4,5) P 2 levels was achieved by densitometry analysis as described in the Methods section, and values are expressed as mean±s.e.m. ( n =6 for WT, n =4 for p110 δ D910A/D910A , n =3 for bovine chromaffin cells, Student's t -test, * P <0.05). ( d , e ) Chromaffin cells were transfected with PH-PLC δ1 -EGFP, and plasma membrane patches were examined by TIRF microscopy at 1 frame per second. Images are displayed in pseudocolour to highlight the changes in fluorescence intensity in the indicated conditions. The images shown were taken from the beginning (left) and peak (right) of the IC87114-induced effect. The insets display the fluorescence intensity change from a selected region of interest on the plasma membrane patches taken at the indicated time points. ( f ) Time-course variation of PH-PLC δ1 -EGFP fluorescence intensity on the (selected) plasma membrane patches in the indicated conditions. ( g ) Average peak fluorescence intensity change of PH-PLC δ1 -EGFP in the respective conditions expressed as mean±s.e.m. (Student's t -test, ** P <0.01). Scale bar, 10 μm. Full size image We next repeated this experiment using bovine chromaffin cells and further tested whether the IC87114-mediated increase in PtdIns(4,5) P 2 could be prevented by preincubation of the cells with the PTEN-specific inhibitor, VO-OHpic. A similar significant increase in PtdIns(4,5) P 2 levels was detected in bovine chromaffin cells treated with IC87114, an effect which was also sensitive to VO-OHpic pretreatment ( Fig. 2c ). We also analysed phosphoinositide levels by high-performance liquid chromatography [25] . Bovine chromaffin cells were 32 P-radiolabelled for 2 h before being treated with either DMSO or IC87114 for 5 min. Phosphoinositides were then extracted, deacylated and analysed on a SAX–HPLC column. IC87114 treatment was found to promote a significant increase (154±9%) of total cellular PtdIns(4,5) P 2 pools compared with vehicle alone ( Supplementary Fig. S2 ). Unfortunately, we could not consistently detect PtdIns(3,4,5) P 3 under our experimental conditions, probably due to the scarcity of the lipid. Consequently, our findings point to a possible role of plasma membrane PTEN in generating PtdIns(4,5) P 2 in response to PI3Kδ specific inhibition, although we cannot exclude the possibility of a parallel contribution from other pathway(s). PtdIns(4,5) P 2 signal induced by p110δ inhibition To gain a deeper insight into the kinetics of the plasma membrane PtdIns(4,5) P 2 generation elicited by IC87114, bovine chromaffin cells were transfected with PH-PLCδ 1 fused to EGFP (PH-PLCδ 1 -EGFP), a specific probe for PtdIns(4,5) P 2 (ref. 26 ) and examined by total internal reflection fluorescence (TIRF) microscopy. The intensity of the PH-PLCδ 1 -EGFP fluorescent signal on the plasma membrane clearly increased in response to IC87114 through cytosolic recruitment ( Fig. 2d ; Supplementary Movie 1 ). Although the increase was detected throughout the examined footprint, local hotspots were observed in which the intensity increase was higher than in other regions of the plasma membrane ( Fig. 2d ). Importantly, IC87114 did not increase PtdIns(4,5) P 2 levels after preincubation of the cells with VO-OHpic ( Fig. 2e–g ; Supplementary Movie 2 ). In an attempt to simultaneously detect the rise in PtdIns(4,5) P 2 and a drop in PtdIns(3,4,5) P 3 , chromaffin cells were transfected with either Akt-PH-GFP or Btk-PH-GFP (PtdIns(3,4,5) P 3 probes) with PH-PLCδ 1 -mRFP. However, both Akt-PH-GFP and Btk-PH-GFP abolished the IC87114-mediated rise in PtdIns(4,5) P 2 and the intensity of their staining at the plasma membrane did not change ( Supplementary Fig. S3 ). One possible explanation could be that sequestration of PtdIns(3,4,5) P 3 prevented the PTEN dephosphorylation of PtdIns(3,4,5) P 3 in response to IC87114 treatment. Alternatively, overexpression of Akt-PH-GFP or Btk-PH-GFP could antagonize PtdIns(3,4,5) P 3 -mediated Akt activation as previously shown [27] , raising the possibility that Akt might be involved in generating the IC87114-mediated rise in PtdIns(4,5) P 2 . Indeed, pretreatment of chromaffin cells with A6730, an Akt inhibitor, blocked this effect ( Supplementary Fig. S4 ). This suggests that PI3Kδ signalling through Akt might contribute to the control of PTEN activity or have a direct effect on PtdIns(4,5) P 2 production. Altogether, our results suggest that PTEN is involved in generating the rise in PtdIns(4,5) P 2 evoked by IC87114, an effect that is regulated by Akt and/or other kinases. More work is required to clarify the mechanism by which IC87114 exerts its effects. IC87114 shifts the release probability to an earlier release Having characterized the nature of the IC87114-mediated PtdIns(4,5) P 2 signal, we next investigated whether the kinetics of exocytotic events was altered by IC87114 using amperometry. We found that IC87114 treatment of chromaffin cells significantly increased the number of exocytotic events occurring during the initial phase of secretion ( Fig. 3a,b ), resulting in an increase in the size of the releasable pool, as previously described [8] . This effect was also blocked by preincubation with VO-OHpic ( Fig. 3c,d ). 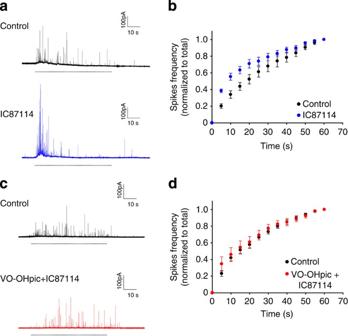Figure 3: IC87114 promotes an increase in the releasable pool size. Mouse adrenal chromaffin cells were stimulated with 70 mM K+solution for 1 min (dotted line below trace), and catecholamine release measured from single cells using carbon fibre amperometry (a, upper trace). Individual current spikes indicate exocytosis from a single vesicle. Pre-incubation of cells with IC87114 (1 μM) for 2 min before stimulation caused a shift in release probability so that more vesicles were released earlier (a, bottom trace). This is quantified in (b) and values expressed as mean±s.e.m. (n=6 cells). (c) Catecholamine release measured using carbon fibre amperometry from a control cell (c, upper trace) and a cell treated with the combination of VO-OHpic (100 nM) and IC87114 (c, bottom trace). Normal secretion was observed in both cases and the treatment did not promote a shift in vesicle release probability compared with earlier time points (d). Data are expressed as mean±s.e.m. (n=8 cells). Figure 3: IC87114 promotes an increase in the releasable pool size. Mouse adrenal chromaffin cells were stimulated with 70 mM K + solution for 1 min (dotted line below trace), and catecholamine release measured from single cells using carbon fibre amperometry ( a , upper trace). Individual current spikes indicate exocytosis from a single vesicle. Pre-incubation of cells with IC87114 (1 μM) for 2 min before stimulation caused a shift in release probability so that more vesicles were released earlier ( a , bottom trace). This is quantified in ( b ) and values expressed as mean±s.e.m. ( n =6 cells). ( c ) Catecholamine release measured using carbon fibre amperometry from a control cell ( c , upper trace) and a cell treated with the combination of VO-OHpic (100 nM) and IC87114 ( c , bottom trace). Normal secretion was observed in both cases and the treatment did not promote a shift in vesicle release probability compared with earlier time points ( d ). Data are expressed as mean±s.e.m. ( n =8 cells). Full size image IC87114 promotes vesicle mobilization and translocation The potentiating effect of IC87114 on exocytosis could stem from an increased priming of vesicles pre-docked and/or from an increased translocation of vesicles to the plasma membrane that, when combined with a Ca 2+ signal, could readily increase the number of vesicles undergoing fusion. To differentiate between these two non-exclusive possibilities, TIRF microscopy was used to image chromaffin cells expressing human growth hormone fused to GFP (hGH–GFP), a marker stored within neurosecretory vesicles. TIRF microscopy is ideal to study vesicle translocation, docking and fusion [28] , as motions in the z -axis can be monitored at high resolution via sensitive changes in fluorescence intensity within an exponentially decaying evanescent wave of excitation light [29] . We investigated motion and intensity of hGH–GFP-positive secretory vesicles in cells treated with IC87114. A significant increase in the number of vesicles undergoing translocation toward the plasma membrane was detected ( Fig. 4a,b ; Supplementary Movie 3 ). The bulk of this translocation was transient and could not be detected in chromaffin cells pretreated with VO-OHpic ( Fig. 4c,d ; Supplementary Movie 4 ). To exclude the possibility of an artifactual increase in fluorescence intensity associated with an overall movement of the cell towards the coverslip, we labelled the plasma membrane of cells expressing neuropeptide Y (NPY)-mCherry (NPY–Cherry) with FITC-tagged wheat germ agglutinin (WGA). This allowed us to confirm that IC87114 promoted translocation of NPY-positive vesicles without causing any significant fluorescence change in WGA-labelled plasma membrane ( Supplementary Fig. S5 ). 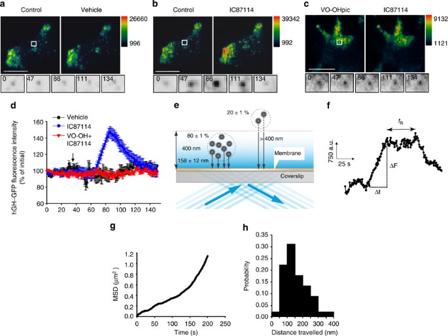Figure 4: IC87114 promotes an active translocation of secretory vesicles to the plasma membrane dependent on PTEN activity. Bovine chromaffin cells expressing hGH–GFP were examined by TIRF microscopy and imaged at 1 frame per second while being treated with either (a) vehicle alone or IC87114 (1 μM) in the presence (b) or absence (c) of VO-OHpic (100 nM). Images taken before and at the peak of treatment are displayed in pseudocolour. A representative example of chromaffin cells from at least three independent experiments is shown. The insets show the fluorescence intensity change of identified vesicles in the above-mentioned conditions. (d) The time-course variations of the overall hGH–GFP fluorescence intensity expressed as a percentage of the initial intensity (n=3–8 randomly chosen regions of interest per condition). (e) Cartoon illustrating the results of the vertical displacement analysis of secretory vesicles in response to IC87114 treatment. The calculation of vesicle displacement to the plasma membrane in the evanescent field was derived from the calibration of the evanescent field (seeMethods). Vesicles not detectable before treatment, but that underwent translocation to the plasma membrane in response to IC87114 (20±1% of the secretory vesicles (n=10 cells)), were excluded from our displacement analysis because of the uncertainty over their original positions. Vesicles that were already present in the evanescent field (~400 nm) were found to travel on average 158±12 nm (n=53 vesicles from 8 cells) to the plasma membrane in response to IC87114 treatment. Note that only vesicles fast approaching and residing on the plasma membrane for more than 10 s (tR>10 s) were taken into consideration to avoid contamination from free-moving vesicles randomly moving towards the plasma membrane without reaching it, as described previously52. (f) Time-course of the fluorescence intensity of a tracked NPY–Cherry-positive vesicle. Changes in fluorescence intensity (ΔF) were used to calculate its penetration depth. (g) Plot of the mean square displacement versus time interval for the tracked vesicle in (f). Note that all the vesicles travelling to the plasma membrane underwent directed motion before reaching the plasma membrane. (h) Probability distribution of the IC87114-induced secretory vesicle displacement to the plasma membrane. Figure 4: IC87114 promotes an active translocation of secretory vesicles to the plasma membrane dependent on PTEN activity. Bovine chromaffin cells expressing hGH–GFP were examined by TIRF microscopy and imaged at 1 frame per second while being treated with either ( a ) vehicle alone or IC87114 (1 μM) in the presence ( b ) or absence ( c ) of VO-OHpic (100 nM). Images taken before and at the peak of treatment are displayed in pseudocolour. A representative example of chromaffin cells from at least three independent experiments is shown. The insets show the fluorescence intensity change of identified vesicles in the above-mentioned conditions. ( d ) The time-course variations of the overall hGH–GFP fluorescence intensity expressed as a percentage of the initial intensity ( n =3–8 randomly chosen regions of interest per condition). ( e ) Cartoon illustrating the results of the vertical displacement analysis of secretory vesicles in response to IC87114 treatment. The calculation of vesicle displacement to the plasma membrane in the evanescent field was derived from the calibration of the evanescent field (see Methods ). Vesicles not detectable before treatment, but that underwent translocation to the plasma membrane in response to IC87114 (20±1% of the secretory vesicles ( n =10 cells)), were excluded from our displacement analysis because of the uncertainty over their original positions. Vesicles that were already present in the evanescent field (~400 nm) were found to travel on average 158±12 nm ( n =53 vesicles from 8 cells) to the plasma membrane in response to IC87114 treatment. Note that only vesicles fast approaching and residing on the plasma membrane for more than 10 s ( t R >10 s) were taken into consideration to avoid contamination from free-moving vesicles randomly moving towards the plasma membrane without reaching it, as described previously [52] . ( f ) Time-course of the fluorescence intensity of a tracked NPY–Cherry-positive vesicle. Changes in fluorescence intensity (ΔF) were used to calculate its penetration depth. ( g ) Plot of the mean square displacement versus time interval for the tracked vesicle in ( f ). Note that all the vesicles travelling to the plasma membrane underwent directed motion before reaching the plasma membrane. ( h ) Probability distribution of the IC87114-induced secretory vesicle displacement to the plasma membrane. Full size image We next attempted to estimate the average displacement of secretory vesicles in the TIRF plane upon IC87114 treatment. The population of vesicles (~20%) that only appeared in the TIRF plane after IC87114 treatment was excluded from our analysis due to uncertainty over their starting positions ( Fig. 4e ). For secretory vesicles that underwent translocation and docking to the plasma membrane ( Fig. 4f,g ), we found that the average distance travelled was 158±12 nm ( Fig. 4h ). To test whether the translocating vesicles undergo partial or full fusion, we used VAMP2-pHluorin, a pH-sensitive form of GFP targeted to the luminal part of secretory vesicles that dequench on exposure to the extracellular environment [28] . Bovine chromaffin cells co-expressing NPY–Cherry and VAMP2-pHluorin, were treated with IC87114. IC87114 promoted a significant translocation of NPY–Cherry to the plasma membrane but no dequenching of VAMP2-pHluorin could be detected ( Supplementary Fig. S6 ; Supplementary Movie 5 ). This suggests that the vesicles mobilized to the plasma membrane undergo transient docking but not fusion. Control experiment of cells treated with IC87114 and further stimulation with barium promoted a significant increase in both NPY–Cherry and VAMP2-pHluorin fluorescent signal intensity ( Supplementary Fig. S6 ; Supplementary Movie 6 ). Actin remodelling is required for vesicle translocation The cortical actin network in chromaffin cells is known to act as a barrier, preventing large dense core vesicles (LDCVs) from accessing the plasma membrane. On Ca 2+ entry, the disruption of the cortical actin cytoskeleton allows access of the secretory vesicles to the plasma membrane [1] . Recently, a more active role of the cytoskeleton has been suggested [3] . We hypothesized that the actin cytoskeleton might act downstream of PtdIns(4,5) P 2 to provide new actin tracks for vesicular transport. We first tested the effect of actin disruption by cytochalasin D, an inhibitor of actin polymerization [29] . Pretreatment of chromaffin cells with cytochalasin D prevented IC87114-mediated hGH–GFP-positive vesicle translocation to the plasma membrane ( Fig. 5a ; Supplementary Movie 7 ) without affecting the PtdIns(4,5) P 2 signal ( Fig. 5b ; Supplementary Movie 8 ). This suggests that actin could have an active role in mediating this IC87114-induced vesicular translocation. 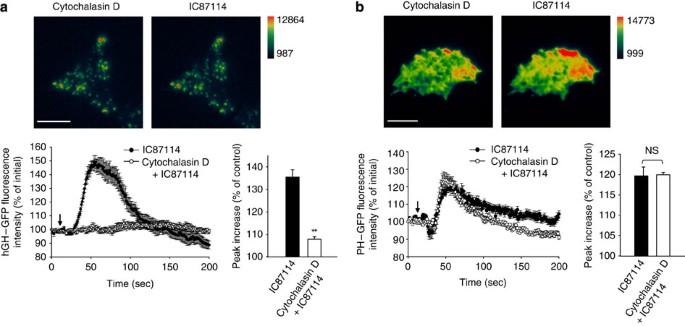Figure 5: Cytochalasin D prevents the IC87114-mediatd secretory vesicle translocation to the plasma membrane. Bovine chromaffin cells expressing (a) hGH–GFP or (b) PH-PLCδ1-EGFP were briefly washed with buffer A before incubation with cytochalasin D (2 μM) for 20 min. Cells were examined by TIRF microscopy and imaged at 1 frame per second before and after the addition of IC87114 (1 μM). The images shown in pseudocolour are taken at the beginning (left) and the peak (right) of the IC87114-induced effect. The time-course of the changes in hGH-GFP or PH-PLCδ1-EGFP fluorescence intensity is expressed as percentage of the initial fluorescence intensity (n=5–7 regions of interest per condition). Average peak fluorescence increases in the indicated conditions are expressed as mean±s.e.m. (n=7 hGH-GFP expressing cells andn=3–5 PH-PLCδ1-EGFP expressing cells. Student'st-test, **P<0.01). Scale bar, 10 μm. Figure 5: Cytochalasin D prevents the IC87114-mediatd secretory vesicle translocation to the plasma membrane. Bovine chromaffin cells expressing ( a ) hGH–GFP or ( b ) PH-PLCδ1-EGFP were briefly washed with buffer A before incubation with cytochalasin D (2 μM) for 20 min. Cells were examined by TIRF microscopy and imaged at 1 frame per second before and after the addition of IC87114 (1 μM). The images shown in pseudocolour are taken at the beginning (left) and the peak (right) of the IC87114-induced effect. The time-course of the changes in hGH-GFP or PH-PLC δ1 -EGFP fluorescence intensity is expressed as percentage of the initial fluorescence intensity ( n =5–7 regions of interest per condition). Average peak fluorescence increases in the indicated conditions are expressed as mean±s.e.m. ( n =7 hGH-GFP expressing cells and n =3–5 PH-PLC δ1 -EGFP expressing cells. Student's t -test, ** P <0.01). Scale bar, 10 μm. Full size image To directly visualize actin tracks, bovine chromaffin cells were transfected with Lifeact–RFP, a peptide capable of binding actin without perturbing its function [30] . Lifeact–RFP was found to co-localize with phalloidin staining of cortical actin ( Fig. 6a ). Nicotine stimulation, which triggers exocytosis by promoting Ca 2+ influx into cells, promotes fragmentation and reorganization of cortical actin ( Fig. 6a , arrows), as previously described [1] , [31] . Lifeact staining of cortical actin visualized on the footprint of a living chromaffin cells revealed a web-like appearance as previously inferred [32] ( Fig. 6b ; Supplementary Movie 9 ). Importantly, Lifeact–RFP expression did not significantly affect the nicotine-induced hGH release from PC12 cells ( Fig. 6c ). Lifeact is, therefore, a suitable marker for imaging F-actin in living neurosecretory cells, which allowed us to investigate the effect of IC87114 on actin by TIRF microscopy. 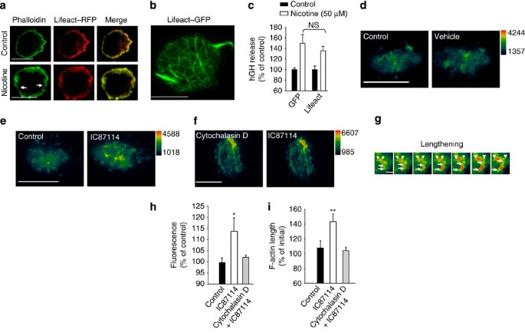Figure 6: IC87114 promotes actin remodelling that is sensitive to cytochalasin D. (a) Untreated and nicotine (50 μM)-stimulated bovine chromaffin cells expressing Lifeact–RFP were fixed and counterstained with phalloidin–FITC. The images shown were taken at the mid-section of chromaffin cells by confocal microscopy. Membrane fragmentations observed after nicotine stimulation are indicated by arrows. (b) Maximum intensity projection of a chromaffin cell expressing Lifeact–GFP on the adherent side of the cell. (c) PC12 cells co-expressing pXGH5 encoding hGH and either GFP or Lifeact–RFP were treated with or without nicotine (50 μM) for 15 min in Buffer A containing 2 mM CaCl2at 37 °C. hGH releases are expressed as mean±s.e.m. (n=3 independent experiments). (d–g) Chromaffin cells expressing Lifeact–GFP (in pseudocolour) were pre-incubated with (f) or without (d,e,g) cytochalasin D (2 μM) for 20 min and imaged by TIRF microscopy at 1 frame per second before and after addition of IC87114 (1 μM). The images shown in pseudocolour are taken at the beginning (left) and the peak (right) of the IC87114-induced effect. (g) Selected regions of growing actin filaments (arrows and arrowheads). Scale bar, 1 μm. (h) Quantification of the average peak increase in Lifeact–GFP fluorescence intensity as a percentage of control (n=5–6 cells per condition). (i) Quantification of F-actin length (n=16–18 from 5 cells). Data are expressed as mean±s.e.m. Student'st-test *P<0.05; **P<0.01. Scale bar, 10 μm. Figure 6: IC87114 promotes actin remodelling that is sensitive to cytochalasin D. ( a ) Untreated and nicotine (50 μM)-stimulated bovine chromaffin cells expressing Lifeact–RFP were fixed and counterstained with phalloidin–FITC. The images shown were taken at the mid-section of chromaffin cells by confocal microscopy. Membrane fragmentations observed after nicotine stimulation are indicated by arrows. ( b ) Maximum intensity projection of a chromaffin cell expressing Lifeact–GFP on the adherent side of the cell. ( c ) PC12 cells co-expressing pXGH5 encoding hGH and either GFP or Lifeact–RFP were treated with or without nicotine (50 μM) for 15 min in Buffer A containing 2 mM CaCl 2 at 37 °C. hGH releases are expressed as mean±s.e.m. ( n =3 independent experiments). ( d – g ) Chromaffin cells expressing Lifeact–GFP (in pseudocolour) were pre-incubated with ( f ) or without ( d , e , g ) cytochalasin D (2 μM) for 20 min and imaged by TIRF microscopy at 1 frame per second before and after addition of IC87114 (1 μM). The images shown in pseudocolour are taken at the beginning (left) and the peak (right) of the IC87114-induced effect. ( g ) Selected regions of growing actin filaments (arrows and arrowheads). Scale bar, 1 μm. ( h ) Quantification of the average peak increase in Lifeact–GFP fluorescence intensity as a percentage of control ( n =5–6 cells per condition). ( i ) Quantification of F-actin length ( n =16–18 from 5 cells). Data are expressed as mean±s.e.m. Student's t -test * P <0.05; ** P <0.01. Scale bar, 10 μm. Full size image Treatment of chromaffin cells with IC87114 promoted an increase in Lifeact–GFP fluorescence by TIRF microscopy ( Fig. 6d,e ). This fluorescence-increase was dependent on actin polymerization as it was blocked by pretreatment with cytochalasin D ( Fig. 6f–i ). This indicates that increased levels of PtdIns(4,5) P 2 are indeed capable of promoting actin remodelling in the immediate vicinity of the plasma membrane. To further examine the relationship between actin remodelling and vesicle translocation, chromaffin cells were co-transfected with Lifeact–GFP and NPY–Cherry to label F-actin and LDCVs, respectively. Vesicles undergoing IC87114-induced translocation were spatially and temporally associated with actin filaments as evidenced in kymographs ( Fig. 7a–c ). 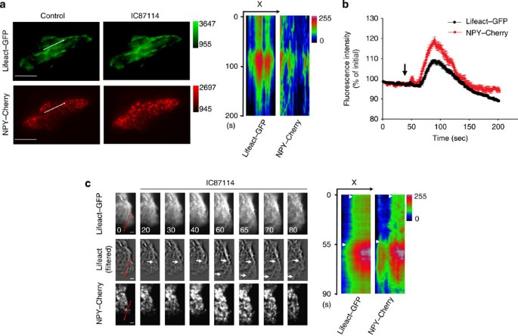Figure 7: IC87114-induced vesicle translocation is correlated with F-actin reorganization. (a) TIRF images (left) and kymographs (right) of bovine chromaffin cells co-expressing Lifeact–GFP and NPY–Cherry treated with IC87114 (1 μM). The scanning lines (white arrows) indicate the position and direction of scan. (b) Time-course variation of Lifeact–GFP and NPY–Cherry fluorescence intensity in response to IC87114 treatment (n=4 regions of interest). The arrow indicates the timing of IC87114 addition. (c) Time-lapse images (left) of selected regions highlighting growing actin filaments and associated vesicle translocation before and during IC87114 treatment. Lifeact–GFP staining was filtered with a Laplacian 2D to highlight edges of actin filaments (middle panel). The timing (in s) after IC87114 treatment is indicated in the series of images. Scale bar, 1 μm. Kymographs (right) illustrate the changes in Lifeact–GFP and NPY–Cherry distribution on the scanning lines (red arrows). Note the increase in NPY–Cherry vesicle intensity occurring near the newly formed actin track. Figure 7: IC87114-induced vesicle translocation is correlated with F-actin reorganization. ( a ) TIRF images (left) and kymographs (right) of bovine chromaffin cells co-expressing Lifeact–GFP and NPY–Cherry treated with IC87114 (1 μM). The scanning lines (white arrows) indicate the position and direction of scan. ( b ) Time-course variation of Lifeact–GFP and NPY–Cherry fluorescence intensity in response to IC87114 treatment ( n =4 regions of interest). The arrow indicates the timing of IC87114 addition. ( c ) Time-lapse images (left) of selected regions highlighting growing actin filaments and associated vesicle translocation before and during IC87114 treatment. Lifeact–GFP staining was filtered with a Laplacian 2D to highlight edges of actin filaments (middle panel). The timing (in s) after IC87114 treatment is indicated in the series of images. Scale bar, 1 μm. Kymographs (right) illustrate the changes in Lifeact–GFP and NPY–Cherry distribution on the scanning lines (red arrows). Note the increase in NPY–Cherry vesicle intensity occurring near the newly formed actin track. Full size image This rapid remodelling of F-actin pointed to the involvement of actin-nucleating factors [33] . As Cdc42 is required for PtdIns(4,5) P 2 -induced actin cytoskeleton remodelling [34] , we transfected chromaffin cells with a WT-Cdc42 or a dominant-negative plasmid (Cdc42-T17N) [35] . Whereas untransfected control cells or expression of WT-Cdc42 did not affect the IC87114-mediated vesicle translocation, Cdc42-T17N completely blocked IC87114-induced vesicle translocation ( Fig. 8a–c ), consistent with a role for Cdc42 in mediating actin reorganization in response to increased PtdIns(4,5) P 2 . To further examine the role of Cdc42 in this process, we directly measured Cdc42 activity in response to IC87114 treatment in chromaffin cells. IC87114 treatment significantly increased Cdc42-GTP levels compared with vehicle-treated cells, demonstrating a small but significant activation of Cdc42 ( Fig. 8d ). We also determined whether Cdc42 activation could occur in living cells using a Cdc42-binding domain (CBD) from WASP that binds specifically to the active form of Cdc42 (ref. 36 ). When chromaffin cells co-expressing CBD–YFP and mCherry, as a marker for cytosol, were treated with IC87114, a recruitment of the domain was detected on specific regions of the plasma membrane ( Supplementary Fig. S7 ). 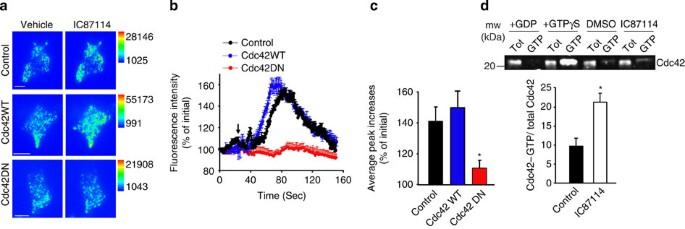Figure 8: IC87114-induced vesicle translocation is dependent on Cdc42. (a) Bovine chromaffin cells expressing NPY–Cherry alone (control) or co-expressing either wild-type Cdc42 or the dominant negative Cdc42(T17N)–GFP (Cdc42DN) construct with NPY–Cherry were visualized by TIRF microscopy. Cells were imaged at 1 frame per second before and after addition of IC87114 (1 μM). The changes in fluorescence intensity of NPY–Cherry are displayed in pseudocolour. The images shown are taken from before the IC87114 treatment and at the peak of its effect. (b) The time-course variations of NPY–Cherry in the indicated conditions are expressed as percentage of the initial intensity. (c) Quantification of the peak fluorescence intensity increases (% of initial) is expressed as mean±s.e.m. (n=3–5 cells per condition). Scale bar, 10 μm. (d) Bovine chromaffin cells treated with DMSO (control) or 1 μM IC87114 (20 min) were lysed and assayed for activated Cdc42 (GTP–Cdc42) by western blotting. Control chromaffin cells were incubated with GDP (negative control) or GTPγS (positive control) and assayed. Bar graph shows the percentage of activated Cdc42 in control and IC87114-treated cells (n=3 independent experiments). Data are expressed as mean±s.e.m. Student'st-test *P<0.05. Figure 8: IC87114-induced vesicle translocation is dependent on Cdc42. ( a ) Bovine chromaffin cells expressing NPY–Cherry alone (control) or co-expressing either wild-type Cdc42 or the dominant negative Cdc42(T17N)–GFP (Cdc42DN) construct with NPY–Cherry were visualized by TIRF microscopy. Cells were imaged at 1 frame per second before and after addition of IC87114 (1 μM). The changes in fluorescence intensity of NPY–Cherry are displayed in pseudocolour. The images shown are taken from before the IC87114 treatment and at the peak of its effect. ( b ) The time-course variations of NPY–Cherry in the indicated conditions are expressed as percentage of the initial intensity. ( c ) Quantification of the peak fluorescence intensity increases (% of initial) is expressed as mean±s.e.m. ( n =3–5 cells per condition). Scale bar, 10 μm. ( d ) Bovine chromaffin cells treated with DMSO (control) or 1 μM IC87114 (20 min) were lysed and assayed for activated Cdc42 (GTP–Cdc42) by western blotting. Control chromaffin cells were incubated with GDP (negative control) or GTPγS (positive control) and assayed. Bar graph shows the percentage of activated Cdc42 in control and IC87114-treated cells ( n =3 independent experiments). Data are expressed as mean±s.e.m. Student's t -test * P <0.05. Full size image Our data therefore support a growing body of evidence that indicates an important role for actin remodelling in order to mobilize and translocate LDCVs to release sites [3] , [35] —a process that we reveal is controlled by PtdIns(4,5) P 2 . Using a combination of pharmacological and genetic manipulations, we have shown that selective inhibition of PI3Kδ leads to a transient increase in PtdIns(4,5) P 2 production, at least partly attributed to the dephosphorylation of PtdIns(3,4,5) P 3 by PTEN. Using this pathway, we found that PtdIns(4,5) P 2 controls the number of secretory vesicles available for exocytosis by regulating vesicular mobilization, translocation and transient docking to the plasma membrane. Our results clearly establish a functional link between PtdIns(4,5) P 2 signalling and secretory vesicle dynamics through de novo remodelling of the actin cytoskeleton mediated by Cdc42 activation. The pan-PI3K inhibitor LY294002 has been shown to exhibit a biphasic effect on secretion [8] : an early phase of potentiation of exocytosis followed by an inhibitory phase, which is correlated with parallel changes in PtdIns(4,5) P 2 levels observed on isolated membrane sheets. Here we have identified a likely mechanism behind the initial rise in PtdIns(4,5) P 2 biphasic effect as being triggered by PI3Kδ inhibition, which prevented new production of PtdIns(3,4,5) P 3 and leading to the dephosphorylation of PtdIns(3,4,5) P 3 by dis-inhibition of PTEN. Consistent with our finding, recent studies have also shown that PI3Kδ can upregulate PTEN, leading to an increase in PtdIns(4,5) P 2 production [19] , [21] . We also investigated other potential sources of the IC87114-mediated rise in PtdIns(4,5) P 2 by examining potential downstream effects of PI3K signalling on Akt activity. Selective inhibition of Akt kinase by A6730 abolished the IC87114-induced PtdIns(4,5) P 2 production. Although it is still unclear how Akt regulates PtdIns(4,5) P 2 production, it is plausible that this could occur either by the activation of PTEN or through an alternative pathway. Interestingly, a reduction in PI3K signalling caused by the loss of the PI3K regulatory unit p85α was shown to reduce PTEN activity [37] , supporting the notion that PI3K signalling (possibly via Akt) could control PTEN activity. Overall, our results are consistent with an effect of PI3Kδ inhibition on PtdIns(4,5) P 2 levels through direct or indirect (Akt-mediated) activation of PTEN. We found evidence of non-homogeneous PtdIns(4,5) P 2 clusters on the plasma membrane as previously described [8] , [38] . Some of these PtdIns(4,5) P 2 clusters were more sensitive to IC87114, as evidenced by a greater increase in PtdIns(4,5) P 2 levels compared with elsewhere on the plasma membrane. This inhomogeneity could result from local conversion of PtdIns(3,4,5) P 3 within PtdIns(4,5) P 2 clusters and/or a non-homogeneous distribution of PTEN/PI3Kδ on the plasma membrane. Our current findings also demonstrate that PI3Kδ is expressed in adrenal chromaffin cells in both early endosomal-containing fractions and the plasma membrane. This isoform could therefore have a role in early endosomal function, as previously suggested for p110β [39] . Importantly, there is an overlap between PTEN and PI3Kδ in the plasma membrane-enriched fractions. PTEN localization on the plasma membrane is regulated by RhoA and RhoA-associated kinase activity [36] and inhibition of PI3Kδ has previously been shown to activate RhoA and RhoA-associated kinase activity [19] . Therefore, PI3Kδ inhibition could potentially promote PTEN recruitment to the plasma membrane and enhance its phosphatase activity, thereby increasing PtdIns(4,5) P 2 levels. Importantly, Myosin 5 also controls PTEN translocation to the plasma membrane in neurosecretory cells and hippocampal neurons [37] . Although our study does not cover the mechanism responsible for PTEN translocation, we detected PTEN in the secretory vesicle fraction, which is also controlled by Myosin-5 (ref. 40 ). Altogether, this points to a role of secretory vesicle exocytosis in delivering PTEN to the plasma membrane, but more work is needed to clarify this issue. The IC87114-mediated increase in PtdIns(4,5) P 2 was sufficient to promote both the active translocation of secretory vesicles to the plasma membrane and, in the presence of stimulation, the fusion of an increased number of secretory vesicles. There is an apparent discrepancy between the transient nature of the effect of PtdIns(4,5) P 2 on actin polymerization and the long-lasting potentiating effect induced by IC87114. Although the mechanism underlying this discrepancy is not clear, it is possible that acute changes in PtdIns(4,5) P 2 levels could not only affect actin polymerization as demonstrated herein, but could also be sufficient to prime a pool of secretory vesicles by signalling through an array of downstream effectors important for priming. In this view, an increase in PTEN activity is likely to stimulate phospholipase D activity [41] thereby promoting the production of phosphatidic acid, a fusogenic lipid critical for the late stages of Ca 2+ -regulated exocytosis in neurosecretory cells [42] . Therefore, the inhibition of PI3Kδ by IC87114 is likely to induce further effects to alter evoked secretion that persist well beyond the transient change observed in PtdIns(4,5) P 2 levels and actin polymerization. Using Lifeact–GFP and TIRF microscopy, we have demonstrated that a rise in PtdIns(4,5) P 2 is sufficient to promote polymerization/remodelling of F-actin in the immediate vicinity of the plasma membrane in neurosecretory cells. Consistent with our findings, expression of PI4P5K Iα has also been shown to induce actin remodelling in COS-7 cells [43] . Hypertonic stress, which increases PtdIns(4,5) P 2 levels by activating PI4 P 5K Iβ, also produces actin polymerization and reorganization [44] . Our finding that 20±1% of vesicles translocate to the plasma membrane from outside the evanescent field following IC87114 treatment, and that vesicles undergoing translocation and transient docking exhibit a directed motion consistent with transport along F-actin, support a growing body of evidence highlighting the role of actin filaments in guiding LDCVs to release sites [3] , [35] . An alternative model for the IC87114-induced vesicular translocation could involve the PtdIns(4,5) P 2 -induced actin polymerization helping to push the vesicles towards the plasma membrane. Due to the short distances travelled by the vesicles originally present in the evanescent field, we are currently unable to conclusively distinguish between the two theories. Cdc42, neural Wiskott–Aldrich syndrome protein and Arp2/3 have been proposed to remodel F-actin, a process that helps to drive neuroexocytosis [3] . Our findings that IC87114 treatment significantly activates Cdc42, and that expression of Cdc42DN inhibits PtdIns(4,5) P 2 -mediated vesicle translocation, indicate that Cdc42 acts as a co-regulator of neural Wiskott–Aldrich syndrome protein [45] to promote local actin polymerization at the plasma membrane. The increased Cdc42 activation could stem from an increase in PtdIns(4,5) P 2 pools and/or a reduction in PtdIns(3,4,5) P 3 concentrations, as previously suggested [46] . In view of the previous finding that Cdc42 facilitates exocytosis in chromaffin cells by stimulating actin polymerization in the vicinity of vesicle docking sites [35] , our data provide a possible link between PtdIns(4,5) P 2 signalling and Cdc42-mediated actin reorganization in the transport of vesicles to the plasma membrane. Although outside the scope of the present study, it would be worth testing whether Myosin-5a could be the actual molecular motor involved in the IC87114-mediated translocation of secretory granules to the plasma membrane [40] . Our estimation of the speed of the translocating vesicles (11.5±1.1 nm s −1 ) is slower than that previously reported for vesicles under depolarization (34±17 nm s −1 ) [28] . One explanation is that the absence of Ca 2+ fails to activate Ca 2+ effectors such as scinderin [47] , which normally contribute to the translocation of secretory vesicles via their loosening effect on the cortical actin network. In conclusion, our results establish a functional link between PtdIns(4,5) P 2 signalling and secretory vesicle translocation to the plasma membrane through the control of cortical actin. Catecholamine release from bovine adrenal chromaffin cells Adrenal chromaffin cells were extracted from adrenal medulla and cultured [48] , [49] . Cells were washed in buffer A (in mM: NaCl, 145; KCl, 5; Na 2 HPO 4 , 1.2; glucose, 10; HEPES–NaOH, 20; pH 7.4) and pre-incubated with the indicated concentrations of IC87114 before being stimulated with or without barium (2 mM) in buffer A. In some cases, cells were stimulated by digitonin (20 μM) permeabilization in KGEP buffer (in mM: K-glutamate, 139; glucose, 5; EGTA, 5; PIPES–NaOH, 20; pH 6.7) containing 2 mM free Mg 2+ , 2 mM ATP and 10 μM free Ca 2+ for 3 min. At the end of each experiment, aliquots of supernatant were taken and the cells were further lysed with 1% (v/v) Triton X-100 (Sigma). Both sets of samples were assayed fluorometrically for catecholamine content. hGH release from transfected PC12 cells PC12 cells were transfected with pXGH5 vector-encoding hGH and indicated constructs for 48 h. Cells were washed and stimulated with or without nicotine (50 μM) in buffer A containing 2 mM CaCl 2 for 15 min before collecting supernatant aliquots. Cells were then lysed with 1% Triton X-100 for measurement of total hGH. The amount of hGH secretion was analysed using an hGH ELISA kit (Roche) according to the manufacturer's instructions. Chromaffin cell labelling Freshly isolated chromaffin cells (4×10 6 cells per well) were transfected by electroporation with the indicated plasmids (2 μg per well) using an Amaxa Rat Neuron Nucleofector Kit (Lonza). After 48–72 h, cells were washed and stimulated with or without nicotine (50 μM) in buffer A containing 2 mM CaCl 2 . They were then fixed with 4% paraformaldehyde for 30 min, washed with PBS and incubated with blocking buffer (0.05% Triton X-100, 0.5% bovine serum albumin (BSA), 3% normal horse serum) for 1 h. Cells were stained with FITC-phalloidin (1 mg ml −1 ) (Sigma) in PBS for 30 min and coverslips mounted with Prolong Gold (Molecular Probes) before being visualized using a LSM 510 confocal microscope (Carl Zeiss). Bovine adrenal medulla fractionation Isolated medulla were homogenized in 0.32 M sucrose in 10 mM Tris, 1 mM EGTA pH 7.4, and subjected to 800 g av centrifugation for 2×15 min. The supernatant was then re-centrifuged for 20 min at 12,000 g av , after which the pellet (12KP) was resuspended in 0.32 M sucrose in 10 mM Tris, 1 mM EGTA pH 7.4 and loaded on a linear sucrose gradient (1M–2.2M) before being centrifuged for 1 h at 100,000 g av . 12×1 ml fractions were collected from the top of the gradient. The supernatant from the 12,000 g av spin (12KSN) was further separated by centrifugation for 1 h at 100,000 g av , after which the pellet and supernatant were collected (100KP and 100KSN). For western blotting, 50 μg of each fraction was solubilized in Laemmli sample buffer and heated for 3 min at 95 °C before loading on an SDS–PAGE gel. Proteins were transferred to Immobilon-FL polyvinylidene difluoride (PVDF-FL) blotting membranes (Millipore) and probed with primary antibodies (anti-p110δ, 1/1,000; anti-PTEN, 1/2,000) and detected using the Odyssey Infrared Imaging System (LI-COR Biosciences) according to the manufacturer's instructions. Rodent adrenal chromaffin cells isolation In each experiment, 4–8 adrenal glands were taken from age-matched adult C57BL/6 mice with approval from the University of Queensland and Flinders University Animal Ethics Committees, and in accordance with the National Health and Medical Research Council of Australia guidelines. The isolated chromaffin cells [44] , [45] were either directly used for lipid analysis or cultured in Dulbecco's modified Eagle's Medium supplemented with 1% penicillin/streptomycin (Invitrogen) and 10% FE tal calf serum (JRH Biosciences) and plated on tissue culture dishes (35 mm, Nunclon) for 3–4 days before experiments. Amperometry Catecholamine release from single chromaffin cells was measured using amperometry [50] by applying +800 mV to a carbon-fibre electrode (ProCFE, Dagan), and recording the resultant current (EPC-9 amplifier and Pulse software, HEKA Electronik), sampled at 10 kHz and low-pass filtered at 1 kHz. Spikes were analysed (Mini Analysis, 6.0.1, Synaptosoft) for a period of 60 s. The bath solution contained 140 mM NaCl, 5 mM KCl, 2 mM CaCl 2 , 1 mM MgCl 2 , 5 mM D -glucose and 10 mM HEPES, pH 7.4. The stimulating solution contained 70 mM K + replacing an equimolar amount of NaCl. Experiments were conducted at 30–32 °C using an in-line solution heater (Warner Instruments). Amperometric spikes were selected, if spike amplitude exceeded 2.5 times the root-mean-squared baseline noise. Cells with 10–200 events were used for the analysis. Lipid extraction and analysis Bovine/mouse chromaffin cells were treated with 1 M HCl at the end of the treatment. Lipids were extracted by the addition of chloroform (CHCl 3 ): methanol (MeOH) (1:1, v/v) and 2 M potassium chloride to the acidified samples. The lower organic phase was collected and dried under a low stream of nitrogen. Dried lipids were resuspended in the lower organic phase and spotted on oxalate-treated TLC plates (Merck). Lipids were separated on TLC plates in a pre-equilibrated glass tank containing CHCl 3 : MeOH: dH 2 0: NH 4 OH (30%) (9:7:1:1 v/v). TLC plates were dried overnight before processing for the overlay assay. For this assay, the TLC plates were blocked in 2.5% BSA (>98% fatty acid free, Sigma) in PBS for 2 h at room temperature. Anti-PtdIns(4,5)P2 antibody 2C11 (2.45 μg ml −1 ; Echelon Biosciences) was added to the blocking buffer for an extra 2 h. Plates were extensively washed with PBS and incubated with anti-mouse HRP-conjugated secondary antibodies (1/500) for 1 h in 1% BSA, washed in PBS and the signal detected using Supersignal West Pico (Pierce). HPLC-based lipid analysis Bovine chromaffin cells were labelled with 0.3 mCi ml −1 inorganic 32 P for 2 h at 37 °C in phosphate-free Dulbecco's modified Eagle's Medium (Invitrogen) supplemented with 10% serum supreme (Lonza) and 10 mM HEPES. Unincorporated 32 P was removed by briefly washing cells with buffer A. Cells were incubated with DMSO or IC87114 (1 μM) for 5 min before the reaction was stopped by placing on ice and the adherent cells removed using a cell scraper. Lipids were extracted by the sequential addition of 96% MeOH/CHCl 3 (2:1, v/v), 3.14% (v/v) Milli-Q water and CHCl 3 containing Folch extract (Sigma) and 2.4 M HCl, 5 mM tetrabutylammonia sulfate. The inorganic phase was collected and dried under vacuum. For deacylation, dried lipids were resuspended in methylamine solution (40% methylamine: butanol: MeOH (42:9:47, v/v/v) and dried at 53 °C in the fume hood. Deacylated samples were then resuspended in 0.5 ml Milli-Q water and extracted with a solution containing butanol/petroleum ether (40–60): ethyl formate (20:4:1, v/v/v). The aqueous phase was collected and dried under vacuum and resuspended in Milli-Q and 32 P-labelled phosphoinositides were separated by HPLC using a partisphere SAX-HPLC column (Whatman, 4.6 mm×125 mm) [25] . Total internal reflection fluorescence microscopy imaging Isolated bovine chromaffin cells were transfected with respective plasmids by electroporation (program X-001) using the Amaxa Rat Neuron Nucleofector Kit (Lonza). Cells were cultured on glass-bottomed culture dishes (MatTek) for 48–72 h before visualizing using a TIRF microscope (Marianas, SDC Everest, Intelligent Imaging Innovations) fitted with a X×100 oil immersion objective (NA=1.46, Zeiss) using an EMCCD camera (QuantEM 512sc). Cells were bathed in buffer A before the addition of IC87114 (Symansis), VO-OHpic (kind gift from Dr. Rudiger Woscholski, Imperial Colleague London), cytochalasin D (Sigma) or A6730 (Sigma) and a time-lapse movie was captured at 1 frame per second for the indicated period. Length of Lifeact–GFP actin fibres was measured using the Slidebook software (version 4.2.0.13). Calibration of evanescent field Fluoresbrite Plain Microspheres (Polysciences) of 2 μm diameter were allowed to settle on the glass-bottom culture MatTek dishes and visualized by TIRF microscopy [51] . The beads located at the glass–water interface were imaged and z-stack TIRF images taken at 0.01 μm interval. Images were analysed to determine the centre of mass of the bead using 2D-Gaussian fitting of the intensity profile using MATLAB (Mathworks). Using the spherical shape of the beads, the distance to the centre of mass was related to the penetration depth of the fluorophore. The exponential decay relationship between fluorescence intensity and the penetration depth was then plotted, and the best fitting parameters were used to estimate the penetration depth ( n =10 beads). Cdc42 activation assay Lysates from bovine chromaffin cultures treated for 20 min with DMSO or IC87114 (1 μM) were assayed for Cdc42 activation using a Cdc42 activation kit, according to the manufacturer's instructions (Millipore). Controls for in vitro GTPγS/GDP loading were prepared by incubation with 1 mM EDTA at 30 °C for 15 min in the presence of 1 mM GDP (negative control) or 100 μM GTPγS (positive control). 10 μg of PAK-1 agarose beads were added to all cleared lysates. Precipitates were washed three times before resuspension in Laemmli sample buffer. Cleared lysates and precipitates from negative and positive controls, DMSO or IC87114 treatments were resolved by SDS–PAGE before western blotting using anti-Cdc42 (1 μg ml −1 ) (Odyssey Infrared Imaging System). Statistical analysis Data analysis was carried out using Student's t -test. All experiments were repeated at least three times. Values are expressed as mean±s.e.m. and data were considered significant at * P <0.05; ** P <0.01. How to cite this article: Wen, P. J. et al . Phosphatidylinositol(4,5)bisphosphate coordinates actin-mediated mobilization and translocation of secretory vesicles to the plasma membrane of chromaffin cells. Nat. Commun. 2:491 doi: 10.1038/ncomms1500 (2011).